Diversity-oriented synthesis as a tool for the discovery of novel biologically active small molecules Small molecular mass chemical entities (so-called small molecules) have always been of interest in chemistry and biology because of their ability to exert powerful effects on the functions of macromolecules that comprise living systems [1] , [2] , [3] . Indeed, the small-molecule modulation of protein function represents the basis for both medicinal chemistry (wherein molecules are sought to chemically modify disease states) and chemical genetics (wherein molecules are used as 'probes' to study biological systems [3] , [4] , [5] , [6] , [7] , [8] . Such chemical modulators are most commonly identified by screening collections or 'libraries' of small molecules. However, a crucial consideration is what compounds to use [3] , [9] , [10] . A general consensus has emerged that library size is not everything; library diversity, in terms of molecular structure and more importantly function, is a crucial consideration. The efficient creation of functionally diverse small-molecule collections presents a formidable challenge. Traditionally, when a specific biological molecule or family of molecules is targeted, the compounds used in the screening process are usually selected or designed on the basis of knowledge of the target structure or the structure of known natural ligands [3] , [9] , [11] . The selection criteria are dramatically complicated if the subsequent screening is 'unbiased'; that is, when the precise nature of the biological target is unknown (for example, in a random drug-discovery screen) [4] , [3] , [12] . In such situations, the structural features required in the small molecules cannot be defined a priori and it can be argued that the screening of a library of compounds that has been designed to interact with one specific biological target (or family of related targets) is not logical, whereas the random screening of many such 'focused' collections can be extremely time and cost demanding. In general, the identification of biologically active small molecules may be aided by screening functionally diverse compound libraries (that is, libraries that display a broad range of biological activities), as it has been argued that a greater sample of the bioactive chemical universe (that is, of all bioactive molecules) increases the chance of identifying a compound with the desired properties [3] , [10] , [13] , [14] . As a corollary, there is a correlation between library functional diversity and the likelihood of identifying small-molecule modulators for a broad range of biological targets in any screening process [10] , [15] . This is particularly important in modern chemical biology studies in which rapid advances in genomic and proteomic approaches to drug discovery are expected to lead to an exponential increase in potential therapeutic targets, creating an ever-increasing demand on access to functionally diverse chemical libraries [10] , [16] . As the biological activity of any given molecule is intrinsically dependent on its structure, the overall functional diversity of a small-molecule library is directly correlated with its overall structural diversity, which in turn is proportional to the amount of chemical space that the library occupies [3] , [10] , [13] . In this review, we comment on various factors associated with efficient creation of functionally diverse small-molecule collections. In particular, we focus on the development of diversity-oriented synthesis (DOS), a synthetic approach that seeks to achieve this goal, primarily through the efficient incorporation of multiple molecular scaffolds in the library. The utility of DOS for the discovery of novel small molecules with exciting biological properties is highlighted. Finally, future perspectives regarding the use and continued development of DOS are discussed. The term 'diversity' is somewhat subjective. Nevertheless, there are four principal components of structural diversity that have been consistently identified in literature [3] , [10] , [12] , [17] , [18] : 1 Appendage diversity (or building-block diversity)—variation in structural moieties around a common skeleton; 2 Functional group diversity —variation in the functional groups present; 3 Stereochemical diversity —variation in the orientation of potential macromolecule-interacting elements; 4 Skeletal (scaffold) diversity —presence of many distinct molecular skeletons. It is worth emphasizing that the overall shape of a small molecule is the most fundamental factor controlling its biological effects. Nature 'sees' molecules as three-dimensional (3D) surfaces of chemical information; a given biological macromolecule will therefore only interact with those small molecules that have a complementary 3D binding surface [1] , [3] , [19] . That is, a given biological macromolecule imposes a degree of shape selection for binding partners; molecules possessing significant shape similarity would thus be expected to generate similar pharmacological responses [20] . The molecular shape diversity of a small-molecule library has therefore been cited as being arguably the most fundamental indicator of overall functional diversity; indeed, substantial 'shape space' coverage (that is, molecular shape diversity) has been correlated with broad biological activity [14] . However, it has been demonstrated that the shape space coverage of any compound set stems mainly from the nature and 3D geometries of the central scaffolds, with the peripheral substituents being of minor importance; that is, the scaffold diversity of a small-molecule library has a pivotal role in defining its overall molecular shape diversity [14] . Scaffold diversity is thus intrinsically linked to shape, and thus functional, diversity. Indeed, there is a widespread consensus that increasing the scaffold diversity in a small-molecule library is one of the most effective ways of increasing its overall structural diversity [3] , [10] , [15] , [19] , [21] and small multiple scaffold libraries are generally regarded as being superior to large single-scaffold libraries in terms of biorelevant diversity [3] , [10] , [14] . Compounds in libraries that are based around different molecular skeletons will display chemical information differently in 3D space, thus increasing the range of potential biological binding partners for the library as a whole [3] . Although there have been advances in the use of computational methods to assess the overall molecular shape diversity of libraries ( vide infra ), the concept of scaffold diversity is arguably more intuitive to a synthetic chemist and is more conveniently related to synthetic accessibility. Therefore, from a DOS perspective, scaffold diversity serves as a useful surrogate measure for shape diversity and thus overall functional diversity. In addition to structural diversity, structural complexity is generally regarded as an important characteristic in small-molecule libraries [3] , [10] , [22] . It has been argued that molecules that are structurally complex are more likely to interact with biological macromolecules in a selective and specific manner [3] , [9] , [10] , [18] , [23] , [24] , [25] . Structurally, and thus functionally, diverse small-molecule libraries should span large regions of biologically relevant chemical space. Consequently, they may prove valuable for the identification of biologically useful small molecules. However, where does one obtain such collections? Broadly speaking, there are three distinct sources of small molecules for use in biological screens: natural products; commercially available compound collections; or new compound collections created by chemical synthesis [3] , [10] . Natural products Numerous natural products have proven to be useful as drugs or leads [26] and nature still represents a major source of innovative therapeutic agents [3] , [10] , [27] . Natural products exhibit enormous structural diversity, including scaffold diversity [3] , [9] , [10] , [28] . However, there are several well-documented problems associated with using natural products in screening experiments (including difficulties with purification, bioactive component identification and chemical modification) [3] , [9] , [10] , [18] , [24] . Commercially available compound collections Commercially available (combinatorial) libraries and pharmaceutical proprietary compound collections represent important alternative sources of molecules [10] . Typically, such collections are comprised of large numbers of structurally simple (generally 'flat') and similar compounds, with 'diversity' limited to variations in appendages attached to a small number of common skeletons [29] . Consequently, the functional diversity (and thus chemical space coverage) achieved by such collections is relatively small. By combining many of these libraries together, a certain degree of chemical diversity can be achieved, such as in the compound archives of large pharmaceutical companies, which typically comprise several million compounds [10] , [18] . However, such corporate compound collections are typically heavily biased towards compounds that satisfy certain predefined criteria imposed by the confines of traditional medicinal chemistry-led optimization campaigns (for example, Lipinski's 'rule of 5' criteria for orally bioavailable drugs) [10] , [23] . This has a number of potential drawbacks, especially in the context of identifying novel bioactive compounds. First, these collections are intrinsically biased towards known bioactive chemical space (that is, the chemical space spanned by known drug molecules and bioactive natural products). Although this is, by definition, a fruitful region for the discovery of biologically useful molecules, it does potentially run the risk of omitting a vast number of bioactive small molecules present in unexplored regions of chemical space from any screening process [1] , [10] . Furthermore, it is likely that the low-hanging fruit within the boundaries of known bioactive chemical space have already been picked [10] . This is particularly important from a business perspective, with crowded intellectual property space an ever-growing problem [30] . Indeed, this is a general disadvantage associated with the use of commercially available compound collections, which are likely to have been thoroughly panned for bioactive constituents. Such deficiencies in current compound collections are evidenced by the continuing decline in drug-discovery successes [30] . Therefore, there is a demand, both from patentability and therapeutic perspectives, for novel biologically active molecules with unusual modes of action that function on underexploited drug targets. Medicinal chemistry research has traditionally been focused around a limited set of biological targets. Indeed, there are only approximately 500 distinct targets of the current pharmacopoeia [29] , [31] . To put this in perspective, the informational content of the human genome has been estimated at around 30,000 genes [31] , [32] . The term 'undruggable' has been coined to describe those biological targets and processes that bear little resemblance to the molecular drug targets exploited in present-day drug therapy and have thus historically been thought of as difficult, if not impossible, to modulate with small molecules [29] , [33] . Human genetics and physiology are increasingly revealing the root causes of human disorders, and this has resulted in validation of several new targets for a range of human diseases [34] , [35] . However, the majority of the relevant targets and processes fall into the 'undruggable' category [29] , [33] , [34] . These include transcription factors, regulatory RNAs, oncogenes and processes such as protein–protein interactions and protein–DNA interactions [29] , [33] . It has been argued that one of the reasons why these processes are traditionally viewed to be impervious to modulation by small molecules is because of deficiencies in existing compound collections (be they pharmaceutical or commercially available). That is, the candidate small molecules that populate many screening collections seem to be well suited to modulating 'traditional' medicinal chemistry targets, but lack the necessary structural elements required to modulate other processes [29] , [33] , [34] , [35] , [36] , [37] . Thus, although vast numbers of compounds from such libraries are frequently screened at great expense, relatively few biologically active 'hits' against these 'undruggable' targets have been found [29] . Therefore, there is a clear need for new small-molecule collections that span regions of bioactive chemical space not accessed by traditional compound libraries in order to identify molecules capable of modulating these more challenging targets ( vide infra ). New compound collections The problems associated with the use of natural products and 'traditional' commercially available combinatorial-type libraries in screening experiments have spurred the development of a variety of synthetic approaches for the de novo creation of small-molecule collections [9] , [10] . Most of these 'modern' methods have abandoned the mass synthesis and screening dogma underpinning early combinatorial chemistry and instead seek to either (1) identify and efficiently access areas of chemical space that have an enhanced probability of containing bioactive compounds or (2) efficiently interrogate wide regions of chemical space simultaneously [3] , [4] , [10] . The former approach is exemplified by methods such as biologically oriented synthesis [38] , biology-inspired synthesis [4] , privileged structure synthesis [39] and diverted-total synthesis [40] , which seek to generate compound libraries based around the core structures of known biologically active molecules, typically natural product templates [10] . The rationale behind this approach is that evolutionary pressure has 'prevalidated' natural products, and thus compounds that are structurally similar, to be able to modulate biological systems [3] , [4] , [10] , [41] . Consequently, it has been argued that such compound libraries should have a high degree of biological relevance, that is, contain a high proportion of biologically active compounds. However, such methods have an intrinsic preencoded scaffold bias and inevitably generate compound collections with a relatively low degree of overall scaffold diversity [10] . Thus, only a relatively small region of total chemical space is covered, with a heavy emphasis towards known bioactive regions [10] . However, what if one wishes to access unexplored regions of chemical space? These areas may contain molecules with exciting, novel biological properties, which interact with new target molecules or function by means of novel modes of action [10] . In particular, there is a demand for compounds with atypical molecular scaffolds. The known universe of organic chemistry is generally dominated by a remarkably small number of molecular scaffolds; for example, in a recent study of known cyclic molecules, 0.25% of the molecular frameworks were found in 50% of known compounds [9] , [42] . This scenario demonstrates a clear need for novel molecular scaffolds to explore and exploit uncharted regions of chemical space [43] . In this context, a less-focused approach is required. The use of non-biased, diversity-driven synthetic approaches, which aim to access a wider range of chemical space by virtue of increased library structural diversity, may thus be more useful [10] . It is widely accepted that it is not synthetically feasible to produce all theoretically stable, small carbon-based molecules [3] , [12] , [23] . Furthermore, making and screening molecules cost, both in terms of time and money [3] , [9] , [10] . Thus, the synthesis of a molecular library that achieves wide coverage of bioactive chemical space presents a formidable challenge to the synthetic chemist; selectivity is an important consideration [3] . The ideal synthesis of a structurally diverse library is one in which this diversity is achieved in the most efficient manner possible [9] . DOS seeks to achieve this goal, primarily through the efficient incorporation of multiple molecular scaffolds in the library. DOS has been defined as the deliberate, simultaneous and efficient synthesis of more than one target compound in a diversity-driven approach [12] . The overall aim of a DOS is to generate a small-molecule collection with a high degree of structural, and thus functional, diversity that interrogates large areas of chemical space simultaneously. This includes known bioactive chemical space (which, by definition, is a fruitful region for the discovery of biologically active agents) and 'un-tapped' regions of chemical space, which may contain molecules with exciting and unusual biological properties that have thus far escaped the attention of humans and perhaps even nature [10] . In principle, the screening of such libraries should provide hits against a range of biological targets, including those typically viewed as being more challenging, with increased frequency and decreased cost [29] . This should yield novel chemical probes for biological research and new drugs for therapeutic interventions [10] . The overall planning strategy of a DOS differs considerably from that used in 'traditional' combinatorial syntheses ( Fig. 1 ). A DOS pathway is analysed in the forward sense; simple starting materials (in this case, a single compound) are converted into a collection of structurally diverse small molecules, usually in no more than five synthetic steps (in order to maximize synthetic efficiency) [1] , [3] , [10] , [12] , [44] . DOS libraries are usually smaller in size compared with commercially available (combinatorial) libraries. However, the molecules are typically structurally more complex, have a greater variety of core scaffolds and possess richer stereochemical variation [10] , [45] . Consequently, the overall structural diversity and thus chemical space coverage achieved in a DOS library is greater ( Fig. 2 ). 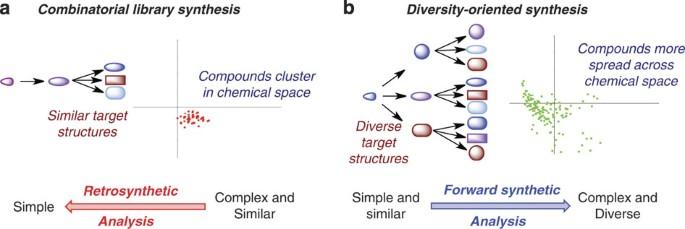Figure 1: Synthetic strategies in combinatorial synthesis and DOS. A comparison of the overall synthetic strategies used in a traditional combinatorial synthesis (a) and a branching DOS pathway (b) (that is, retrosynthetic or forward synthetic analysis), together with a visual representation of the chemical space coverage achieved (that is, focused around a specific point or diverse coverage)3,10,18. Figure 1: Synthetic strategies in combinatorial synthesis and DOS. A comparison of the overall synthetic strategies used in a traditional combinatorial synthesis ( a ) and a branching DOS pathway ( b ) (that is, retrosynthetic or forward synthetic analysis), together with a visual representation of the chemical space coverage achieved (that is, focused around a specific point or diverse coverage) [3] , [10] , [18] . 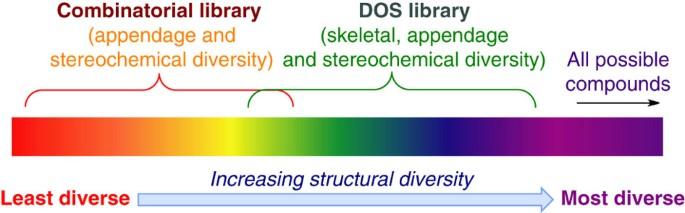Figure 2: The molecular diversity spectrum. In qualitative terms, 'diversity' can be viewed as a spectrum ranging from a target-oriented synthesis of one specific molecule to the synthesis of all possible molecular entities (that is, total chemical space coverage). A traditional combinatorial approach and a DOS will produce compound collections between these two extremes. It should be the goal of a DOS to synthesize, in a qualitative sense, collections as near as possible to the right-hand side of the spectrum3,10,18. Full size image Figure 2: The molecular diversity spectrum. In qualitative terms, 'diversity' can be viewed as a spectrum ranging from a target-oriented synthesis of one specific molecule to the synthesis of all possible molecular entities (that is, total chemical space coverage). A traditional combinatorial approach and a DOS will produce compound collections between these two extremes. It should be the goal of a DOS to synthesize, in a qualitative sense, collections as near as possible to the right-hand side of the spectrum [3] , [10] , [18] . Full size image A successful DOS must address the four principal types of structural diversity mentioned previously [1] , [4] , [18] , [44] , [46] . The most challenging facet of DOS, and of central importance to its success, is the ability to efficiently incorporate skeletal diversity into a compound collection [1] , [3] , [9] , [10] , [19] , [47] , [48] . The efficient generation of multiple molecular scaffolds is regarded as one of the most effective methods of increasing the overall structural diversity of a collection of molecules and has been reported to increase the odds of addressing a broad range of biological targets (relative to a single-scaffold library) [3] , [9] , [10] , [14] , [15] , [18] , [19] , [49] . The process of varying functional group, appendage and stereochemical diversity around privileged scaffolds is occasionally referred to as 'DOS around a privileged scaffold' [35] . However, we believe that the true ethos of DOS is based around a diverse, non-focused coverage of chemical space, which is most efficiently achieved though variation in all aspects of diversity, including skeletal. In this context, we are of the opinion that the term 'DOS around a privileged scaffold' is somewhat of a contradiction in terms, and other descriptions are more appropriate for the process of library generation around a privileged scaffold ( vide supra ). However, it should be emphasized that such an approach is a perfectly valid means of identifying new biologically active small molecules and may be particularly useful in more target-biased biological screens. There are two principal approaches towards generating skeletal diversity in a DOS context, the reagent-based approach and the substrate-based approach ( Fig. 3 ) [1] , [3] , [10] , [30] , [50] . The reagent-based approach is a branching synthetic strategy that involves the use of a common starting material and different reagents [3] , [10] . A short series of divergent, complexity-generating reactions is carried out on the starting material to produce a collection of compounds with distinct molecular skeletons [1] , [3] , [10] . The substrate-based approach to skeletal diversity is based around a folding process and involves the use of different starting materials and common reaction conditions. A collection of substrates that contain appendages with suitable 'preencoded' skeletal information (so-called σ elements) into products have distinct molecular skeletons using a common set of conditions ( Fig. 3 ) [1] , [3] , [10] , [48] , [50] . In practice, such methods are usually based around intramolecular reactions that 'pair' strategically positioned functional groups in the substrates, resulting in compounds with diverse skeletons [3] , [10] , [30] . 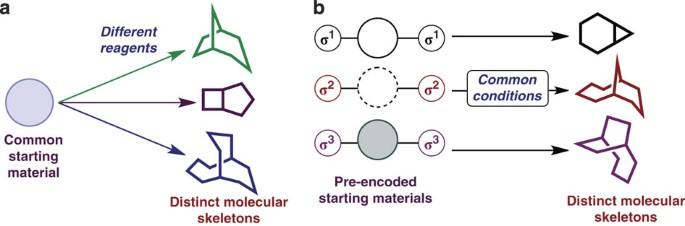Figure 3: DOS approaches to scaffold diversity. (a) The reagent-based approach to scaffold diversity. (b) The substrate-based approach to scaffold diversity3,10. A σ element is an appendage on a starting material that 'pre-encodes' skeletal information (that is, a skeletal information element) such that, under a certain set of reaction conditions, a product containing a different, distinct molecular skeleton is generated19. Figure 3: DOS approaches to scaffold diversity. ( a ) The reagent-based approach to scaffold diversity. ( b ) The substrate-based approach to scaffold diversity [3] , [10] . A σ element is an appendage on a starting material that 'pre-encodes' skeletal information (that is, a skeletal information element) such that, under a certain set of reaction conditions, a product containing a different, distinct molecular skeleton is generated [19] . Full size image It should be noted that a given DOS pathway may incorporate both branching and folding-type reactions, but from the point of view of skeletal diversity construction, the overall strategy used will generally fall into one of the two general categories outlined above (for example, reagent-based pathways for skeletal diversity generation typically incorporate folding reactions as discrete steps). Illustrative representative examples of diversity-oriented syntheses using reagent- and substrate-based approaches for the generation of scaffold diversity are given below. In practice, reagent-based skeletal diversity is achieved using two main methods [1] , [3] , [10] , [18] : 1 The use of a densely functionalized molecule in which different functionalities in the same molecule are transformed by different reagents (that is, pairing different parts of the same densely functionalized molecule); 2 The use of a pluripotent functional group (that is, one that can participate in a number of different reactions) in which exposure of a given molecule to different reagents results in different reactions occurring at the same part (functional group) of the molecule. In both cases, building block, stereochemical and functional group diversity can be introduced into the final library through variation in the substrates used (or, in the case of stereochemical diversity, also through the use of stereoselective reactions) [3] . Reagent-based DOS using densely functionalized molecules An elegant example of this approach is provided by the recent work of Pizzirani et al [34] . The authors have reported the synthesis of a skeletally and stereochemically diverse small-molecule collection by a DOS approach based around the varied reactivity of densely functionalized chiral amino propargylic alcohols 1a–d ( Fig. 4 ). These could be synthesized as a complete matrix of stereoisomers using simple coupling reactions and readily available building blocks. Work focused on the syn - and anti -diastereoisomers 1a , b (on the basis of symmetry, the authors expected that the same reactions would work analogously on enantiomers 1c , d , providing products in all stereochemical combinations, that is, stereochemical diversity). Skeletal diversification was achieved by intramolecular cyclization reactions initiated by reagent- and substrate-controlled site-selective activation of different pairs of functional groups strategically placed around this liner template. 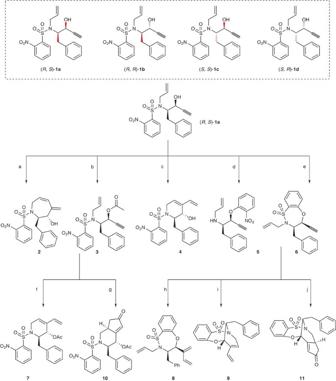Figure 4: A reagent-based DOS pathway. Conditions developed by Pizziraniet al.34: (a) Hoveyda-Grubbs' second-generation catalyst, ethylene, toluene, room temperature (rt); (b) acetic anhydride, triethylamine, dimethylaminopyridine, CH2Cl2, 0 °C; (c) InCl3, 1, 2-dichloroethane, microwave 90 °C; (d) tetra-n-butylammonium fluoride, tetrahydrofuran (THF), 0 °C; (e) NaH, THF, −10 °C; (f) Hoveyda-Grubbs' second-generation catalyst, ethylene, CH2Cl2, 45 °C; (g) [CO2(CO)8], trimethylamineN-oxide, THF, rt; (h) Hoveyda-Grubbs' second-generation catalyst, ethylene, benzene, rt; (i) Hoveyda-Grubbs' first-generation catalyst, CH2Cl2, rt then Pb(OAc)4; (j) [CO2(CO)8], trimethylamineN-oxide, THF, rt. Figure 4: A reagent-based DOS pathway. Conditions developed by Pizzirani et al . [34] : (a) Hoveyda-Grubbs' second-generation catalyst, ethylene, toluene, room temperature (rt); (b) acetic anhydride, triethylamine, dimethylaminopyridine, CH 2 Cl 2 , 0 °C; (c) InCl 3 , 1, 2-dichloroethane, microwave 90 °C; (d) tetra- n -butylammonium fluoride, tetrahydrofuran (THF), 0 °C; (e) NaH, THF, −10 °C; (f) Hoveyda-Grubbs' second-generation catalyst, ethylene, CH 2 Cl 2 , 45 °C; (g) [CO 2 (CO) 8 ], trimethylamine N -oxide, THF, rt; (h) Hoveyda-Grubbs' second-generation catalyst, ethylene, benzene, rt; (i) Hoveyda-Grubbs' first-generation catalyst, CH 2 Cl 2 , rt then Pb(OAc) 4 ; (j) [CO 2 (CO) 8 ], trimethylamine N -oxide, THF, rt. Full size image Initially, a series of five diversification reactions were carried out on 1a , yielding products 2–6 with four new molecular scaffolds generated ( Fig. 4 ). These reactions were based around reactivity at four of the different functionalities present in 1a , that is, the hydroxyl group, the alkene, the alkyne and the amine moieties: (1) enyne metathesis (route a); (2) acylation (route b); (3) indium-mediated skeletal rearrangement (route c); (4) Smiles rearrangement (route d); and (5) sodium hydride-mediated intramolecular cyclization (route f). Further skeletal diversification of compounds 3 and 6 was achieved by methathesis reactions (routes f, h and i), which yielded products 7–9 , and cobalt-mediated Pauson–Khand reactions (routes g and j) that generated products 10 and 11 . The net result was that this DOS strategy enabled the synthesis of a collection of single-isomer small molecules the members of which displayed appendage, functional group, stereochemical and skeletal diversity, with around 14 different molecular skeletons being present among the molecules produced. Other examples of the use of a densely functionalized molecule strategy to generate scaffold diversity in a DOS context can be found in recent reports and reviews [18] , [51] , [52] , [53] , [54] . Reagent-based DOS using a pluripotent functional group strategy A pluripotent DOS is dependent on the use of a synthetically versatile starting material that is capable of undergoing a wide variety of different chemical transformations and has the potential to be converted into several products with different molecular skeletons through the variation of reagents alone [3] . These products should themselves contain versatile functionality and thus be suitable for further diversification, preferably in further complexity-generating and branching reaction sequences. This provides a means to augment the skeletal diversity of the library further and ideally offers scope for the introduction of stereochemical diversity [3] . An example of scaffold diversity generation using a pluripotent functional group is provided by the work of Thomas et al [55] . This DOS involved the use of solid-supported phosphonate 12 as a starting unit ( Fig. 5 ) [3] . The imidazolidinone portion of 12 (R group in Fig. 5 ) allowed the attachment of compounds at each stage of the synthesis to a novel silyl-polystyrene solid support resin [56] , which simplified purification during library synthesis. 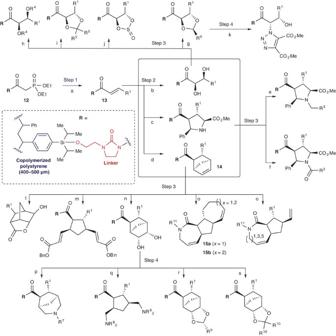Figure 5: DOS of 242 compounds based of 18 discrete molecular frameworks. Conditions: (a) LiBr, 1,8-diazabicyclo[5.4.0]undec-7-ene, R1CHO, MeCN; (b) AD-mix-α, THF/H2O (1:1); (c) (R)-QUINAP, AgOAc,iPr2NEt, α-imino-ester, THF, −78 °C to 25 °C; (d) chiral bis(oxazoline), Cu(OTf)2, 3 Å MS, CH2Cl2, C5H6; (e) R3CHO, BH3-pyridine, MeOH; (f) R2COCl, DMAP, pyridine, CH2Cl2; (g) R6CHO, TsOH, DMF, 65 °C; (h) R4Br, Ag2O, CH2Cl2, 40 °C; (i) R5C(O)R5, TsOH, DMF, 65 °C; (j) SOCl2, pyridine, CH2Cl2, 40 °C; (k) NaN3, DMF, 100 °C then DMAD, toluene, 65 °C; (l)mCPBA, CH2Cl2then MeOH, 65 °C; (m) CH2=CHCO2Bn, Hoveyda-Grubbs' second-generation catalyst, ethylene, toluene, 120 °C; (n) OsO4, NMO, CH3C(O)CH3/H2O (10:1); (o) RNH2, Me2AlCl, toluene 120 °C; then NaH, R11X, DMF, THF; then toleune, 120 °C, Hoveyda-Grubbs' second-generation catalyst, ethylene; (p) NaIO4, THF/H2O (1:1); then R7NH2, NaB(OAc)3H, CH2Cl2; (q) NaIO4, THF/H2O (1:1); then R8NHR8, NaB(OAc)3H, CH2Cl2; (r) R9CHO, DMF, TsOH, 60 °C; (s) R10C(O)R10, DMF, TsOH, 60 °C. DMAD, dimethyl acetylenedicarboxylate; DMF, dimethyl formamide; THF, tetrahydrofuran. Figure 5: DOS of 242 compounds based of 18 discrete molecular frameworks. Conditions: (a) LiBr, 1,8-diazabicyclo[5.4.0]undec-7-ene, R 1 CHO, MeCN; (b) AD-mix-α, THF/H 2 O (1:1); (c) ( R )-QUINAP, AgOAc, i Pr 2 NEt, α-imino-ester, THF, −78 °C to 25 °C; (d) chiral bis(oxazoline), Cu(OTf) 2 , 3 Å MS, CH 2 Cl 2 , C 5 H 6 ; (e) R 3 CHO, BH 3 -pyridine, MeOH; (f) R 2 COCl, DMAP, pyridine, CH 2 Cl 2 ; (g) R 6 CHO, TsOH, DMF, 65 °C; (h) R 4 Br, Ag 2 O, CH 2 Cl 2 , 40 °C; (i) R 5 C(O)R 5 , TsOH, DMF, 65 °C; (j) SOCl 2 , pyridine, CH 2 Cl 2 , 40 °C; (k) NaN 3 , DMF, 100 °C then DMAD, toluene, 65 °C; (l) m CPBA, CH 2 Cl 2 then MeOH, 65 °C; (m) CH 2 =CHCO 2 Bn, Hoveyda-Grubbs' second-generation catalyst, ethylene, toluene, 120 °C; (n) OsO 4 , NMO, CH 3 C(O)CH 3 /H 2 O (10:1); (o) RNH 2 , Me 2 AlCl, toluene 120 °C; then NaH, R 11 X, DMF, THF; then toleune, 120 °C, Hoveyda-Grubbs' second-generation catalyst, ethylene; (p) NaIO 4 , THF/H 2 O (1:1); then R 7 NH 2 , NaB(OAc) 3 H, CH 2 Cl 2 ; (q) NaIO 4 , THF/H 2 O (1:1); then R 8 NHR 8 , NaB(OAc) 3 H, CH 2 Cl 2 ; (r) R 9 CHO, DMF, TsOH, 60 °C; (s) R 10 C(O)R 10 , DMF, TsOH, 60 °C. DMAD, dimethyl acetylenedicarboxylate; DMF, dimethyl formamide; THF, tetrahydrofuran. Full size image The first step of DOS (Step 1, Fig. 5 ) involved E -selective Horner–Wadsworth–Emmons reactions of 12 with a variety of aldehyde building blocks (building block diversity) to deliver 12 α,β-unsaturated acyl-imidazolidinones 13 [3] . In the second step of DOS (Step 2), the pluripotent nature of 13 was exploited in three catalytic enantioselective divergent reaction pathways (stereochemical diversity), namely, (1) (2+3) cycloaddition (reaction b); (2) dihydroxylation (reaction c); and (3) (4+2) cycloaddition (reaction d), to furnish molecules on the basis of three molecular frameworks (skeletal diversity) [3] . The next step of DOS (Step 3) involved a series of branching reactions to further diversify these substrates. For example, the norbonene derivatives 14 served as versatile substrates for a series of branching reactions (reactions l to o) to create five different molecular scaffolds (skeletal diversity). Of particular note was an interesting tandem ring-closing-opening-closing metathesis reaction (reaction o) that generated skeletally diverse tricyclic products 15a (7-5-7) and 15b (7-5-8) [3] . A fourth stage of reactions (Step 4) was carried out in some cases to introduce additional complexity and diversity. In the final step of the DOS (not shown), the compounds were cleaved off the solid support using a variety of reagents (appendage diversity) [3] . Using the chemistry shown in Figure 5 and a limited number of structurally diverse building blocks, a DOS of 242 small molecules was achieved, which have 18 molecular frameworks among other unique structural features. Many of these frameworks have no known representation in nature, highlighting the capability of this DOS approach to generate products that populate new, unexplored regions of chemical space [3] . Other examples of the use of a pluripotent functional group strategy to generate scaffold diversity in a DOS context can be found in recent reports and reviews [18] , [49] . The substrate-based approach The substrate-based approach towards scaffold diversity is exemplified in a recent DOS pathway developed by Morton et al . [57] ( Fig. 6 ). Their method involved the attachment of pairs of unsaturated functionalized building blocks (so-called 'propagating' and 'capping' groups) to a fluorous-tagged linker to generate a wide variety of substrates with a dense array of structural features (appendage, functional group and stereochemical diversity) [9] . Each of these substrates contained a pair of terminal alkene groups (one from the linker, one from the 'capping' building block), together with additional unsaturated moieties. Treatment with a suitable metathesis catalyst led to intramolecular cyclization reactions that 'paired' these unsaturated functional groups together to generate a dense matrix of skeletally diverse cyclic products [9] . The elegant design of the fluorous-tagged linker ensured that only cyclized products were released from the fluorous tag during the metathesis process. Consequently fluorous solid-phase extraction provided a rapid, generic method for product isolation [9] . The overall result was the DOS of a library of 96 molecules (each generated in no more than five discrete steps) based on a total of 84 distinct molecular scaffolds. The compounds can be considered to be natural product-like, in the sense that a diverse range of different 3D features and functionalization motifs are present (stereochemical and functional group diversity). It is noteworthy that the majority of library scaffolds ( ∼ 65%) are novel. This work arguably represents the current state of the art for scaffold diversity generated in a synthetic small-molecule library. 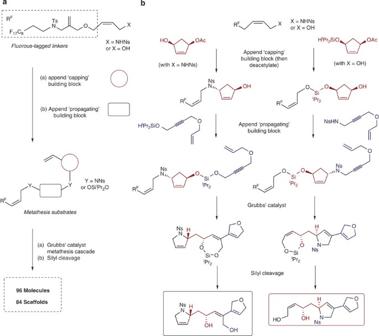Figure 6: A substrate-based DOS approach. (a) Outline of the synthetic route used by Mortonet al.57for library synthesis9,57. (b) Two representative examples of scaffold diversity generation. For precise details regarding conditions, the reader is directed towards the primary text57. Figure 6: A substrate-based DOS approach. ( a ) Outline of the synthetic route used by Morton et al . [57] for library synthesis [9] , [57] . ( b ) Two representative examples of scaffold diversity generation. For precise details regarding conditions, the reader is directed towards the primary text [57] . Full size image The build-couple-pair strategy Recent work by Nielsen and Schreiber [30] has identified a common strategic feature that is present in many DOS pathways. 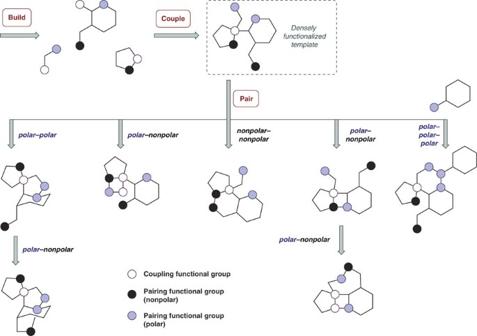Figure 7: Generation of skeletal diversity with a build/couple/pair strategy. The three phases can be defined in the following manner:build: asymmetric syntheses of chiral building blocks; couple: intermolecular coupling reactions that join the building blocks are performed; this process provides the basis for stereochemical diversity;pair: intramolecular coupling reactions that join pairwise combinations of functional groups incorporated in the 'build' phase are performed (polar functional groups marked in blue; nonpolar in black); this process provides the basis for skeletal diversity30. This is the so-called build/couple/pair (B/C/P) three-phase strategy that is outlined in Figure 7 (ref. 30 ). The pair 'phase' is a folding-type process that provides the basis for the generation of skeletal diversity. Figure 7: Generation of skeletal diversity with a build/couple/pair strategy. The three phases can be defined in the following manner: build : asymmetric syntheses of chiral building blocks; couple: intermolecular coupling reactions that join the building blocks are performed; this process provides the basis for stereochemical diversity; pair : intramolecular coupling reactions that join pairwise combinations of functional groups incorporated in the 'build' phase are performed (polar functional groups marked in blue; nonpolar in black); this process provides the basis for skeletal diversity [30] . Full size image For example, the DOS pathway outlined in Figure 4 can be analysed in terms of a B/C/P strategy. The 'build' and 'couple' phases involve assembly of amino alcohols 1a–d . The subsequent reagent-controlled skeletal diversification reactions serve as 'pair' phases in which different combinations of the moieties of a substrate (for example, 1a ), both polar and nonpolar, are 'paired' in functional group-specific reactions. For example, the ruthenium-based catalyst selectively pairs the nonpolar alkene and alkyne groups of 1a , enabling the metathesis reaction leading to 2 , whereas sodium hydride-mediated endocyclic nucleophilic aromatic substitution selectively pairs the polar functional groups to form 6 . In the case of the DOS pathway of Morton et al . [57] ( Fig. 6 ), the 'build' phase involves the synthesis of the 'propagating' and 'capping' building blocks, the 'couple' phase involves the formation of the metathesis substrates and the 'pair' phase involves intramolecular cyclization reactions. It has been argued that the modular nature of syntheses that are based around B/C/P strategy should facilitate both systematic modification and optimization of the resulting products [30] . From a synthetic perspective, the central aim of DOS is the efficient creation of structural diversity and complexity. These considerations place a number of demands on the chemistries appropriate for use in a DOS context. To ensure synthetic efficiency, DOS is dependent on reliable, and usually high-yielding, reactions. Furthermore, the synthetic methodologies used in a DOS must work on a wide variety of substrates and be compatible with a wide range of functional groups. This generally means the use of a known methodology that has a literature precedent. In addition, reactions that are capable of rapidly assembling complex molecular skeletons and generating complex functionalization motifs, such as pericyclic, cascade, multicomponent [58] and tandem reactions, are particularly valuable [35] . Folding-type DOS processes typically exploit the remarkable utility of ring-closing metathesis to generate complex molecular scaffolds from much simpler substrates [9] , [35] , [57] . Although DOS libraries are smaller in size than those resulting from combinatorial-type methods, compound purification still represents a significant bottleneck in the synthesis process. Towards this end, many DOS strategies have used phase-labelling techniques (for example, solid-phase synthesis [55] and fluorous-based tags [49] , [57] ) that facilitate product isolation and purification [11] . One of the criticisms that is commonly levelled at DOS is that the method adds little to the understanding and development of synthetic chemistry. It is indeed true that DOS is dependent on robust reactions, which generally means the use of 'standard' tried-and-tested synthetic methodologies. In this sense, DOS is no different from any other chemical synthetic process that involves a sequence of reactions, such as the conversion of simple starting materials into a specific, more complex target structure, for example, a total synthesis. However, similar to endeavours in the field of total synthesis often leading to fundamental advances in synthetic organic chemistry, so may DOS also serve as an exciting platform for the development of new methodologies and mechanistic understanding [35] . A fundamental issue when attempting the synthesis of a 'diverse' small-molecule library is the subjective nature of diversity itself; that is, how can one compare the overall diversity present in different collections [59] ? Towards this end, numerous computational methods have been developed that seek to assess the diversity of different molecular libraries in a more quantitative manner [40] , [42] , [59] , [60] , [61] . The goal of these methods is not to provide an absolute measure of diversity, but a relative measure that also agrees to a good extent with chemical intuition [3] . For example, some groups have used a computational process for diversity assessment based around the calculation of molecular descriptor values followed by principal component analysis [3] , [53] , [62] . In essence, this provides a measure of total chemical space coverage. Other commonly used methods include the calculation of normalized principle moment-of-inertia ratios for the assessment of molecular shape diversity [34] , [51] and comparison of the polar surface areas of molecules in the library (the polar surface area is a key feature in terms of ligand–receptor binding; indeed, diverse biological activity has been associated with small molecules with diverse polar surface areas) [51] . Recently a computer-based tool called ' Scaffold Hunter ' has been developed which extracts the molecular scaffolds present in a compound collection and correlates the relationship between them in a hierarchical tree-like arrangement [63] , [64] . Not only does this allow a more quantitative, less-subjective assessment of the scaffold diversity contained within a particular chemical collection [57] , [65] , but 'virtual scaffolds' that do not exist in the data set yet that occupy intermediate positions are also constructed in silico and added. 'Brachiation' along the branches from larger more complex scaffolds to smaller scaffolds may lead to less-complex compound classes with the same types of activity [63] . It is important to emphasize the fact that the ultimate success of any small-molecule library is determined by the biological relevance of the compounds it contains [3] , [9] , [10] . If the library does not yield hits in a chosen biological screening experiment, it will be deemed to be unsuccessful, no matter how structurally diverse it is or how efficiently this diversity has been accessed [3] , [10] . In this context, the validity of the DOS approach has been verified by the discovery of numerous novel, biologically active small molecules through the screening of DOS libraries. Significantly, this includes hits against so-called 'undruggable' targets and processes, which have traditionally been seen as difficult or even impossible to modulate with small molecules. Molecules capable of modulating protein–protein interactions [66] , [67] , [68] , transcription factor activity [69] , [70] and multidrug resistance in pathogens [55] , [71] have all been discovered through the use of DOS libraries. 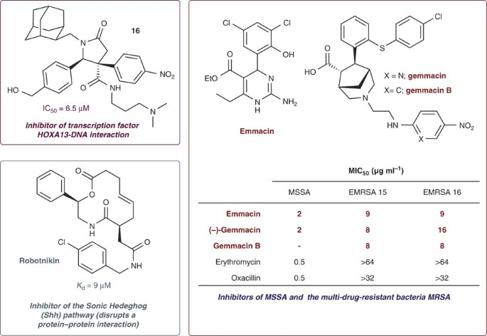Figure 8: DOS and the discovery of biologically active molecules. Some examples of biologically active molecules identified through the screening of DOS libraries (16(ref.69), Robotnikin68, emmacin71, gemmacin55, gemmacin-B84). MSSA, methicillin-susceptibleStaphylococcus aureus; MRSA, methicillin-resistantS. aureus. EMRSA-15 and EMRSA-16 are the two MRSA strains85responsible for the majority of MRSA infections in the United Kingdom and both are resistant to penicillin and erythromycin86. MIC50, minimum inhibitory concentration required to inhibit the growth of 50% of organisms. IC50, half maximal inhibitory concentration (concentration of an inhibitor that is required for 50% inhibition of its target).Kd, dissociation constant. Some examples are shown in Figure 8 . Such results not only validate the usefulness of DOS as a tool for the discovery of novel biologically active small molecules but also illustrate that DOS is capable of addressing some of the limitations associated with more 'typical' small-molecule collections (for example, commercial of pharmaceutical proprietary). Figure 8: DOS and the discovery of biologically active molecules. Some examples of biologically active molecules identified through the screening of DOS libraries ( 16 (ref. 69 ), Robotnikin [68] , emmacin [71] , gemmacin [55] , gemmacin-B [84] ). MSSA, methicillin-susceptible Staphylococcus aureus ; MRSA, methicillin-resistant S. aureus . EMRSA-15 and EMRSA-16 are the two MRSA strains [85] responsible for the majority of MRSA infections in the United Kingdom and both are resistant to penicillin and erythromycin [86] . MIC 50 , minimum inhibitory concentration required to inhibit the growth of 50% of organisms. IC 50 , half maximal inhibitory concentration (concentration of an inhibitor that is required for 50% inhibition of its target). K d , dissociation constant. Full size image In recent years, there has been a significant paradigm shift in the selection criteria for compound libraries used in biological screening experiments, with molecular diversity considerations having an increasingly prominent role [10] . It has been argued that structurally diverse small-molecule libraries should contain compounds with a broad range of biological activities capable of modulating a wide variety of biological processes [29] . DOS has emerged as a synthetic approach that aims to address the formidable challenges associated with the efficient de novo generation of structurally diverse small-molecule libraries. Since Schreiber's seminal works on DOS [1] , [19] , [72] , [73] , [74] , the field has evolved rapidly and diversity-oriented syntheses are growing in number and sophistication. There are numerous examples of novel, biologically useful small molecules that have been discovered through the screening of DOS libraries [10] . This includes hits against 'challenging' biological processes for which 'traditional' libraries usually fail to provide suitable leads or even hits ( vide supra ) [66] . Therefore, it is reasonable to argue that the development of diversity-driven synthetic approaches such as DOS represents significant advancements in the field of chemical biology, offering a potentially powerful approach for the identification of novel molecules with exciting biological properties. Despite the proven utility of DOS for the discovery of novel bioactive small molecules, there remains significant scope for improvement if the full potential of such diversity-driven approaches is to be fulfilled. This includes addressing issues associated with both the synthesis and screening of the small-molecule library. From a synthetic perspective, increasing the efficiency of diversity construction represents an ongoing challenge of great importance. In this context, a crucial consideration is the overall number of synthetic steps required to generate each unique scaffold in the library (so-called step-to-scaffold efficiency [65] ). An inherent drawback of a substrate-based (folding) DOS approach is the requirement for a collection of substrates to be synthesized before the scaffold diversity-generating step (however, the modular nature of such syntheses unquestionably facilitates systematic modification of the resulting products) [9] . Perhaps the ultimate in efficient scaffold generation would be a branching synthetic pathway whereby every single reaction carried out on one simple starting would result in a different molecular scaffold [9] . An additional area that needs to be addressed is the generation of structural complexity in DOS pathways [9] . In many diversity-oriented syntheses, particularly those using a substrate-based approach for scaffold diversity generation, the majority of the complexity and functionality of the final compounds is already present in the starting substrate(s). A crucial question from the point of view of synthetic efficiency is whether it is possible to more efficiently couple scaffold diversity generation with the creation of molecular complexity, such that little of the desired final functionality needs to be present in the starting substrates [9] , [10] . Such challenges are formidable and can only be addressed by the continued development of new synthetic methodologies of broad utility and efficiency. This should reduce our dependency on the limited number of tried-and-tested diversity-generating reaction types typically used in library synthesis and allow access to atypical yet complex structural motifs in a more efficient manner. In addition to synthesis factors associated with DOS, library screening is an area that requires further development. The aim of DOS is to produce a library of molecules with a broad range of biological activities. To fully capitalize on this potentially high level of biodiversity, such collections should, ideally, be screened in every available biological assay, covering as many different biological targets and processes as possible. This presents a significant technical and financial challenge. The ready availability of extensive biological screening facilities has traditionally been a preserve of the private sector. However, recent years have witnessed significant developments in the screening capacity available to public sector researchers, stimulated by advancements in both chemistry and biology and facilitated by increased collaboration between scientists from a wide range of disciplines. Indeed, publicly funded initiatives such as the Broad Institute Chemical Biology Platform [75] and the Sloan-Kettering Institute [76] have been established, with the aim of creating multidisciplinary research environments in which high-throughput capabilities in both organic synthesis and small-molecule screening can be integrated efficiently 'in-house'. The resulting data are typically made accessible to the global community (see, for example, PubChem [77] and the Molecular Libraries Roadmap [78] ). It is envisioned that such broad dissemination should facilitate both the discovery and optimization of new bioactive small-molecule agents. Although such new research centres are undoubtedly valuable, 'traditional' academic institutions remain the mainstay of fundamental biological and chemical research in the public sector. However, despite the obvious benefits associated with well-integrated synthesis-screening facilities, chemical biology studies in many academic institutions remain rather fractured. There needs to be a concerted effort in these situations to develop such an infrastructure, which requires increased interdepartmental and cross-disciplinary collaboration. In addition, the smaller budget available for such studies in traditional academic centres (and indeed, more specialized collaborative institutions or initiatives) relative to industry imposes more stringent limitations on throughput and resources. Consequently, versatile screening platforms are valuable [79] . Furthermore, it may be beneficial for academia to focus its resources on research that avoids direct competition with industry. Areas that may not be profitable enough to warrant investigation by private companies can still be explored in an academic context in which financial gain is not the most important consideration. This can even include therapeutically important fields, such as the discovery of new antibacterials, which have been largely neglected by industry ( vide supra ) [3] . One area that should benefit from the ability of DOS to efficiently generate scaffold diversity is that of fragment-based drug discovery. In most pharmaceutical organizations, traditional screening typically attempts to evaluate as many compounds as technologically possible (typically, a million or more) in the hopes of finding relatively potent drug leads (with K d values ideally less than 1 μM) [80] . Fragment-based drug design is based on screening smaller numbers (typically several thousand) of small-molecule 'fragments' (typically containing less than 18 heavy atoms and a molecular mass no greater than 250 Da) in the hopes of finding low-affinity hits (with K d values in the high micromolar to millimolar range) [80] , [81] . This then reveals core templates that form key interactions with portions of a target binding site. Subsequent elaboration of the fragment can then introduce interactions and compound features that provide the required affinity and selectivity while conventional medicinal chemistry considerations optimize drug-like properties [81] . As with any screening approach, library design is a critical consideration in order to ensure that relevant hits of sufficiently high quality can be obtained [81] , [82] . Small fragments have an increased probability of binding to a given target than do larger, more complex molecules [83] ; increased molecular complexity (and size) reduces the probability of finding leads, because the decoration of compounds increases the chance that useful interactions will not be made by randomly chosen ligands [81] . Therefore, one of the principal advantages of the fragment-based approach is the potential for identifying new chemotypes that unexpectedly satisfy the features of the target binding site [81] . In this context, fragment libraries may benefit from high levels of structural diversity rather than being biased towards a particular compound class [81] , [83] . DOS may be especially valuable for the efficient creation of such collections. Biologically active compounds are the ultimate goal of any small-molecule library synthesis. Thus, a DOS should aim to efficiently and specifically access known and unknown biologically relevant chemical space, rather than chemical space that cannot provide biologically useful molecules [10] . That is, although novel and unusual molecules are desirable, it is still important that they be natural product-like and drug-like in terms of their capability to interact with, and thus modulate, biological systems [3] , [10] . The structural constraints that this consideration imposes on molecules are not precisely known, as the true boundaries of biologically relevant chemical space have yet to be defined (if indeed it is ever possible to do so) [10] . It is generally acknowledged, however, that some improvement in our understanding of the boundaries of biologically relevant chemical space can, and indeed urgently, needs to be achieved; the ability to predict (and thus factor-in during synthesis) the biological relevance of compound libraries is a crucial consideration in terms of the overall efficiency of the synthesis and screening sequence [29] . This is by no means an easy task and will require significant developments in our understanding of the relationship between the structural features of small molecules and screening outcomes [10] , [29] . In this context, the broad dissemination of small-molecule screening data through initiatives such as PubChem [77] is valuable ( vide supra ). On a related note, it is important to remember that the dictates of molecular recognition of a small molecule may vary greatly between different types of molecular targets. For example, it is generally believed that the physiochemical requirements for small molecules against antibacterial targets, protein–protein interactions and central nervous system targets are very different [35] . Some have therefore suggested that more 'focused' DOS libraries, designed with a particular type of molecular target in mind, will be valuable. However, defining the level of structural bias in such a context is, at the moment, somewhat arbitrary and may lend itself to possibly 'excessive' levels of structural conservatism. There always remains the possibility that compounds in regions of chemical space beyond the predefined limits will display activity against the chosen target, perhaps through novel, unexpected (yet potentially exciting) modes of action. Towards this end, Schreiber has argued that the ultimate goal in library synthesis is a 'super-set' of compounds of such structural diversity that, for any given aspect of biological process, members can be found to modulate that aspect [29] . Although this remains a distant (and perhaps ultimately unattainable) dream, the continued evolution of diversity-driven synthetic approaches such as DOS undoubtedly represents steps in the right direction. How to cite this article: Galloway, W.R.J.D. et al . Diversity-oriented synthesis as a tool for the discovery of novel biologically active small molecules. Nat. Commun. 1:80 doi: 10.1038/ncomms1081 (2010).